A double bond with weak σ- and strong π-interactions is still a double bond 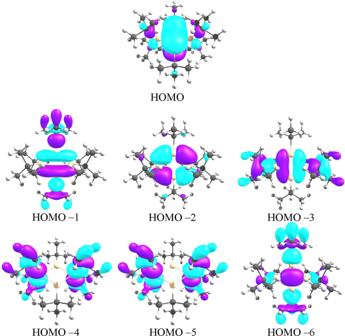Fig. 1: Occupied molecular orbitals. Occupied molecular orbitals of2; HOMO −6 corresponds to a σ-bond across the ring. 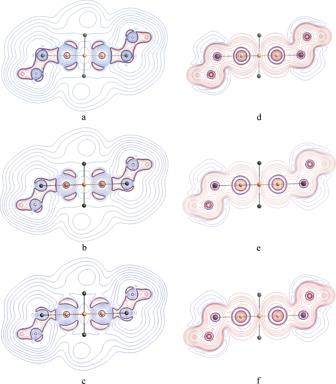Fig. 2: Topology of the derivitives of the electron density. Topology of the derivitives of the electron density; contour plots of the Laplacian of electron density (a–c) and energy density (d–f) in2. CH3groups are removed for more clarity in the plot. Positive and negative values are represented by blue and red lines, respectively.aThe central region between 1,3 atoms has a positive Laplacian that is a sign of closed-shell interaction.bBy removing electrons from the σ-bonding HOMO −6 the electron density concentrations, corresponding to thep-atomic orbitals on the Si atoms intensifies.cRemoving all electrons from the σ-framework of Si4intensifies thep-electron density concentration.dContour plot of energy density that shows a covalent-type interaction between Si atoms.eContour plot of energy density after removing electrons from HOMO −6, and (f) after removing electrons from all σ-MOs of Si4moiety. The p-atomic orbital-shaped feature appears on the Si atoms by removing the σ-electrons in the contour plot of energy density too. The structure of the molecule was taken from the Supplementary Information of the original paper by Kyushin et al. [4] and reoptimized at two levels of theory, B3LYP/6-31g(d) as the original paper (Table S1 ) and B3LYP/def2-TZVP (Table S2 ) for more accuracy by Gaussian 16 [20] . No symmetry was imposed during optimization. A local minimum with lower energy compared to the previously reported structure was found and confirmed via frequency computations. The stability of the wavefunction was examined and the system was found to be stable at the selected computational level. The Si 4 framework keeps its planar structure with D 2h symmetry in the new conformer that allows one to separate σ- and π-frameworks by removing electrons from the corresponding MOs within the framework of Bader’s theory. CMOs of the molecule were analyzed at both levels of theory and no difference was found. The wavefunctions were analyzed and visualized by AIMAll [21] at both levels of theory. The values reported here are from B3LYP/6-31g(d) akin to those reported in the original paper. To evaluate the effect of each MO on bond characteristics, occupation of the corresponding MO in the WFX files was nullified and the bonding analyses repeated. The difference between the magnitude of each parameter in the original wavefunction and the manipulated one provides the effect of the manually unoccupied MO on the desired properties. To compute individual π- and σ-contributions to the DI, the occupation number of the π-MO was nullified. It is worth noting that removing electrons from the σ-framework is not recommended because the σ-electrons constitute the backbone of the electron density and removing them can change the topology of atoms and affect the magnitude of DI [14] , [22] .